Omnidirectional spin-wave nanograting coupler Magnonics as an emerging nanotechnology offers functionalities beyond current semiconductor technology. Spin waves used in cellular nonlinear networks are expected to speed up technologically, demanding tasks such as image processing and speech recognition at low power consumption. However, efficient coupling to microelectronics poses a vital challenge. Previously developed techniques for spin-wave excitation (for example, by using parametric pumping in a cavity) may not allow for the relevant downscaling or provide only individual point-like sources. Here we demonstrate that a grating coupler of periodically nanostructured magnets provokes multidirectional emission of short-wavelength spin waves with giantly enhanced amplitude compared with a bare microwave antenna. Exploring the dependence on ferromagnetic materials, lattice constants and the applied magnetic field, we find the magnonic grating coupler to be more versatile compared with gratings in photonics and plasmonics. Our results allow one to convert, in particular, straight microwave antennas into omnidirectional emitters for short-wavelength spin waves, which are key to cellular nonlinear networks and integrated magnonics. Metamaterials [1] , [2] are artificial materials engineered to gain properties that may not be observed in nature. Photonic crystals [3] , [4] and magnonic crystals (MCs) [5] , [6] , [7] are two examples of metamaterials. They offer enhanced control of light (photons) and spin waves (SWs; magnons), respectively, provoked by periodic patterning at the nanoscale. Bicomponent MCs, formed by periodic alternations of two constituent ferromagnetic materials [8] , [9] , are known to provide an artificially tailored band structure for plane-wave SWs. Forbidden frequency gaps near Brillouin zone boundaries were indeed evidenced in a two-dimensional (2D) Py/Co MC comprising Co nanodisks embedded in thin Ni 80 Fe 20 (Py) films [10] , [11] . In spintronics, a magnetic nano-oscillator (NO) excited by the spin transfer torque (STT) has been shown to act as a point-like source of short-wavelength SWs at GHz frequency [12] , [13] , [14] . The SWs allow one to phase-lock two neighbouring NOs [15] , [16] , [17] . In photonics, directional SW emission has been achieved very recently by external laser sources using specially focused light beams. The relevant wavelengths λ were about 250 (ref. 18 ) and 1.6 μm (ref. 19 ). For parallel processing in magnetic cellular nonlinear networks (CNNs), SWs with small λ are essential [20] . Stimulated by the perspective of novel non-charge-based interconnections and logical devices, magnonics has already entered the international technology roadmap for semiconductors [21] . However, how to convert GHz microelectronics into emitters for short-wavelength plane waves poses unresolved challenges. Micropatterned microwave antennas such as coplanar waveguides (CPWs) [22] emit, for example, micrometre-wavelength SWs in only a limited manner. In photonics and plasmonics, nanoscale grating couplers have been proven to be powerful to control the propagation of light [23] , [24] , [25] , [26] , [27] . In ref. 28 , the idea of converting a microwave field into SWs with a non-magnetic silver grating was introduced. However, the uniform spin-precessional mode with wave vector | k |=2 π / λ =0 was pronounced and partly obscured SWs of shorter wavelength with small signal strength. In this article, we demonstrate multidirectional emission of short-wavelength SWs with large amplitudes from straight microwave antennas. For this, we have created ferromagnetic structures with periodically modulated magnetic properties. The wavelength and propagation direction of the SWs are found to be precisely controlled by reciprocal-lattice vectors G of the periodic structure. The spin-precessional amplitudes of grating-coupler-induced modes are found to be giantly enhanced compared with the original excitation strength of the microwave antennas. Different gratings applied to one-and-the-same microwave antenna allow one to emit plane-wave SWs in any in-plane direction, suggesting the term ‘omnidirectional’. Our results on SW grating couplers represent a unique functionality and will lead to marked advances in SW-based spintronic devices. Magnetic gratings and spectroscopy The SWs are created by an intrinsic magnonic grating-coupler effect in periodically patterned ferromagnets of different dimensionality ( Fig. 1a–d ). 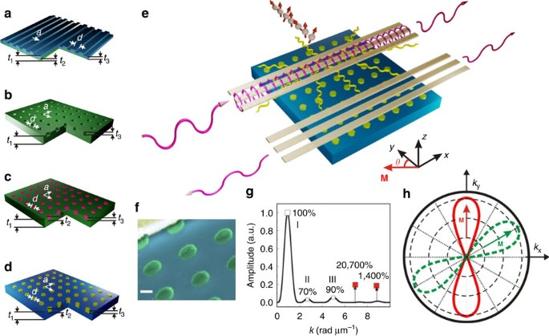Figure 1: Magnonic grating couplers provoking giantly enhanced spin waves. (a) One-dimensional device consisting of periodic Py nanowires (green) coated with CoFeB (blue). (b) 2D lattice consisting of periodic nanotroughs in Py (green). (c) BGC with Co nanodisks embedded in a Py thin film. (d) BGC with Py nanodisks embedded in a CoFeB thin film. (e) CPW integrated to a BGC, where we illustrate the omnidirectional SW excitation (yellow arrows). (f) Coloured scanning electron microscope image taken under a tilt angle of 54° such that nanodisks appear as ellipses. Scale bar, 200 nm. (g) Excitation spectrumI(k) obtained by Fourier transformation of the CPW microwave magnetic field. Squares indicate measured signal strengths. The data are obtained on the BGC witha=800 nm in an in-plane field. Signal strengths are normalized toI(k) in a way considering an excitation efficiency of 100% atkI(largest peak). Empty squares represent modes excited directly by the CPW. Solid squares stand for the grating-coupler-induced modes atkI−G01andkI+G01, showing a giantly enhanced amplitude. (h) Isofrequency contours. Red and green curves are typical isofrequency curves in magnonics when the magnetizationMof an isotropic ferromagnet points in two different directions as indicated. The bold black circle indicates an isofrequency contour in photonics for an isotropic material (for qualitative comparison). An amplitude enhancement is experimentally observed, crucially decided by the artificial lattice patterns, lattice constants and magnetic materials ( Table 1 ). We will focus mainly on 2D CoFeB/Py bicomponent lattices, where Py nanodisks were embedded into a shallow-etched antidot lattice (ADL) prepared from a CoFeB thin film ( Fig. 1e,f ). The nanodisks formed a 2D periodic lattice of lattice constant a with a squared unit cell. We integrated straight micropatterned CPWs to excite and detect SWs ( Fig. 1e ) using a connected vector network analyser (VNA) [29] . The field around the central conductors exerted a torque on the magnetization M . The Fourier analysis of this microwave field provided us with an excitation spectrum I ( k ) (ref. 30 ; Fig. 1g ), which contained three prominent peaks I, II and III at wave vectors k I , k II and k III , respectively. The uniform spin-precessional mode at k =0 was not excited. The reflection data were measured when the SWs were emitted and detected on the same CPW, whereas the transmission data were taken when we excited SWs at one CPW and then detected them on the neighbouring one. Signal lines were separated by s =12 μm (compare Fig. 7 in Methods section). The VNA detected the voltage in a phase-sensitive manner, providing real and imaginary (Im) parts of the signal. The VNA-based technique allowed us to study standing and propagating SWs in wide regimes of frequency and magnetic field H . From each data set, we subtracted a reference spectrum where resonances were shifted away from the relevant frequency regime by an appropriate H to enhance the signal-to-noise ratio for SW excitations. Figure 1: Magnonic grating couplers provoking giantly enhanced spin waves. ( a ) One-dimensional device consisting of periodic Py nanowires (green) coated with CoFeB (blue). ( b ) 2D lattice consisting of periodic nanotroughs in Py (green). ( c ) BGC with Co nanodisks embedded in a Py thin film. ( d ) BGC with Py nanodisks embedded in a CoFeB thin film. ( e ) CPW integrated to a BGC, where we illustrate the omnidirectional SW excitation (yellow arrows). ( f ) Coloured scanning electron microscope image taken under a tilt angle of 54° such that nanodisks appear as ellipses. Scale bar, 200 nm. ( g ) Excitation spectrum I ( k ) obtained by Fourier transformation of the CPW microwave magnetic field. Squares indicate measured signal strengths. The data are obtained on the BGC with a =800 nm in an in-plane field. Signal strengths are normalized to I ( k ) in a way considering an excitation efficiency of 100% at k I (largest peak). Empty squares represent modes excited directly by the CPW. Solid squares stand for the grating-coupler-induced modes at k I − G 01 and k I + G 01 , showing a giantly enhanced amplitude. ( h ) Isofrequency contours. Red and green curves are typical isofrequency curves in magnonics when the magnetization M of an isotropic ferromagnet points in two different directions as indicated. The bold black circle indicates an isofrequency contour in photonics for an isotropic material (for qualitative comparison). Full size image Table 1 Magnonic grating couplers and grating-coupler-induced spin-wave enhancement. Full size table Evidence of grating-coupler modes In the spectra, we find numerous additional modes at large wave vectors k , which evidence backfolding of thin-film dispersion relations f(k) via reciprocal-lattice vectors G . These vectors G point in different spatial directions, even along the CPW. Depending on the geometry and materials, modes reach a signal enhancement as high as ~20,000% compared with the original CPW excitation at the relevant k ( Fig. 1g ). None of these modes is observed in the unpatterned reference sample. The magnonic grating coupler effect enlarges considerably the coupling efficiency between the long-wavelength electromagnetic waves and short-wavelength SWs. The 2D periodic magnetic lattices, that is, the magnetic bi-grating couplers (BGCs), thereby convert a straight microwave antenna into an all-electrical omnidirectional SW emitter, which can be straightforwardly integrated into microwave electronics, CNNs and magnonic applications. A unique characteristic of magnonics is the pronounced anisotropy [31] for SW propagation in an isotropic ferromagnet ( Fig. 1h ). Isofrequency lines in reciprocal space do not form a circle in contrast to photonics when light propagates in an isotropic optical medium [32] . The isofrequency lines in Fig. 1h have been extracted from the thin-film dispersion relations f(k) calculated by the formalism of refs 31 and 33 . In particular, the isofrequency contours in magnonics rotate when one changes the direction of the magnetization M (angle θ , see Fig. 1e ) using an in-plane magnetic field H (ref. 31 ). To evidence the omnidirectional SW emission by the magnonic grating-coupler effect, we make use of the high frequency (energy) resolution of the VNA and the angular dependencies of SW resonances in particular. In Fig. 2a , we plot SW spectra taken at an applied field of 40 mT at different angles θ . Modes k I , k II and k III , generated by the CPW, are observed in both the plane-film and BGC sample with a =800 nm (black and red curves, respectively). These modes are marked with open black squares and arrows. Two further modes (compare also Fig. 7 in Methods section) at higher frequency (over 15 GHz) are detected in the magnetic BGC sample (filled squares) but not in the plane film. Each of the modes shifts towards a smaller resonance frequency with decreasing field angle θ . To illustrate this, we show grey-scale plots for spectra taken at 40 mT on the plane-film sample varying θ from −90° to 200° in Fig. 2b . We resolve the three modes k I , k II and k III depending characteristically on θ and exhibiting different intensities. We now show how this observation is consistent with angular-dependent dispersion relations ( Fig. 3 ) [31] . These relations f(k) allow us to quantify the wave vector k and understand the high-frequency (HF) modes provided by the grating-coupler effect. Using the formalism of ref. 33 , we have modelled the dispersion relations f(k) for different θ . From Fig. 3 , we see that for constant k the measured frequency should vary characteristically as a function of θ (dashed vertical lines). The variation in f is larger for larger | k |. In Fig. 2b , we plot the corresponding angular dependencies quantitatively considering this continuous variation in angle θ between M and k I , k II and k III (dotted lines). For wave vectors k I , k II and k III , we find that the eigenfrequencies measured at θ =90° fall on the Damon–Eschbach (DE) mode dispersion relation of the unpatterned film (solid lines in Fig. 2c and uppermost curve in Fig. 3 ). At θ =90°, the magnetization vector M is perpendicular to k I , k II and k III . We observe a one-to-one correspondence between the relative intensities measured at k I , k II and k III , and the three excitation maxima in I ( k ) of the CPW ( Fig. 1g ). Rotating M to θ =0° and 180°, the three modes in Fig. 2b are found to take their minimum frequencies. These minimum frequencies are consistent with backward volume magnetostatic SWs (BVMSW), where M is collinear with k ( Fig. 3 ). In Fig. 2d , we show the grey-scale data set taken on the BGC sample. Here we highlight the two additional HF modes by red colour. They are of strikingly larger signal strength compared with modes k II and k III . The two modes HF are clearly observed over a wide magnetic field regime (compare Fig. 7 in Methods section). Both modes have their highest resonance frequency f when the field is applied at 90°. Here, f goes down gradually to 5 GHz at 0° and 180°. This angular dependence is similar to the ones of modes excited directly by the CPW at k I , k II and k III . The similarity indicates that these two HF modes exhibit fixed wave vectors k being collinear with k I , k II and k III . At the same time, the large eigenfrequencies at θ =90° evidence large | k | values ( Fig. 3 ). Considering these dispersion relations for DE modes, now we attribute the two HF modes to two modes that are back-folded into the first Brillouin zone of the BGC. The relevant reciprocal-lattice vector G 01 =(0,2 π / a ) (dashed lines in Fig. 2c ) gives rise to excitations at k I + G 01 and k I − G 01 falling onto the dispersion relations in Fig. 2c . On the basis of these wave vectors, we remodel quantitatively the field dependencies of the HF modes in Fig. 2d (dashed lines). 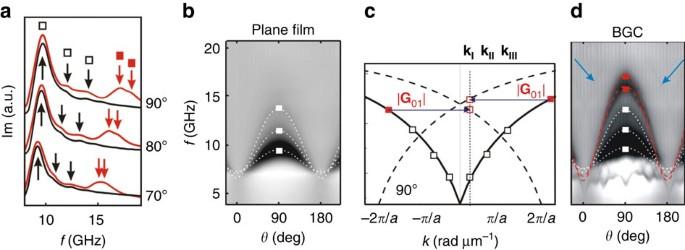Figure 2: Angular-dependent spin-wave spectroscopy and back-folded dispersion relation. (a) Spectra at applied field anglesθ=90°, 80° and 70° measured in reflection configuration. Red (black) curves are data of the BGC (plane film). White and red squares indicate maxima. We note that these line plots are consistent with the data in the grey-scale plots (b) and (d) at respective angles. (b) Grey-scale plot of the spectra such as the ones inataken for differentθon the plane film at 40 mT. White dotted lines represent fittings according to ref.33for the CPW modeskI,kIIandkIII. White squares highlight the resonance frequencies of these three modes atθ=90°. (c) Calculated dispersion relationf(k) of DE modes at 40 mT in a CoFeB plane film atθ=90° for positive and negativek(solid lines). White and red squares are taken from the experimental data ofaat 90°. Red empty squares indicate modes back-folded by ±G01from red solid squares. (d) Grey-scale plot of the angle-dependent reflection signal measured on the BGC with lattice constanta=800 nm. White dotted lines and white squares are the same as inb. The red dashed lines represent calculated angular dependencies for spin-wave modes assumingk=kI+G01(uppermost line) andkI−G01(second highest line). Arrows mark further modes attributed to the grating-coupler effect. Figure 2: Angular-dependent spin-wave spectroscopy and back-folded dispersion relation. ( a ) Spectra at applied field angles θ =90°, 80° and 70° measured in reflection configuration. Red (black) curves are data of the BGC (plane film). White and red squares indicate maxima. We note that these line plots are consistent with the data in the grey-scale plots ( b ) and ( d ) at respective angles. ( b ) Grey-scale plot of the spectra such as the ones in a taken for different θ on the plane film at 40 mT. White dotted lines represent fittings according to ref. 33 for the CPW modes k I , k II and k III . White squares highlight the resonance frequencies of these three modes at θ =90°. ( c ) Calculated dispersion relation f ( k ) of DE modes at 40 mT in a CoFeB plane film at θ =90° for positive and negative k (solid lines). White and red squares are taken from the experimental data of a at 90°. Red empty squares indicate modes back-folded by ± G 01 from red solid squares. ( d ) Grey-scale plot of the angle-dependent reflection signal measured on the BGC with lattice constant a =800 nm. White dotted lines and white squares are the same as in b . The red dashed lines represent calculated angular dependencies for spin-wave modes assuming k = k I + G 01 (uppermost line) and k I − G 01 (second highest line). Arrows mark further modes attributed to the grating-coupler effect. 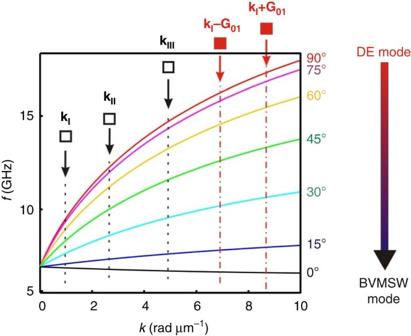Figure 3: Angular dependence of spin-wave dispersion relationsf(k). We showf(k) for seven selected anglesθbetweenMandk. The uppermost (bottom) curve represents a DE (BVMSW) mode. The vertical lines are searching lines for angular-dependent resonance frequencies at differentk-values. Black squares and red squares represent the CPW modes and grating-coupler modes, respectively, consistent with the symbols inFig. 2. Full size image Figure 3: Angular dependence of spin-wave dispersion relations f ( k ). We show f ( k ) for seven selected angles θ between M and k . The uppermost (bottom) curve represents a DE (BVMSW) mode. The vertical lines are searching lines for angular-dependent resonance frequencies at different k -values. Black squares and red squares represent the CPW modes and grating-coupler modes, respectively, consistent with the symbols in Fig. 2 . Full size image SW emission in non-high-symmetry directions A detailed inspection of Fig. 2d reveals further modes (arrows), which follow different angular dependencies compared with the five modes discussed so far. Interestingly, these two modes show maximum eigenfrequencies of about 18.5 GHz near θ =45° and 135°, and undergo crossings at about 15 GHz near 0° and 180°. In Fig. 4a , we summarize the resonance frequencies of these two modes as extracted from the experimental data of Fig. 2d . When we calculate angular dependencies assuming wave vectors k I ± G 11 and k I ± G 1(−1) with | (compare Fig. 4b ), these curves quantitatively remodel the further two modes within the experimental error. 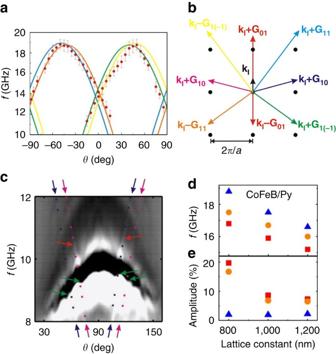Figure 4: Multidirectional spin-wave detection for different BGCs. (a) Data extracted fromFig. 2dfor branches highlighted by arrows. Error bars stand for the line width of the resonance. Blue, orange, green and yellow lines are the fittings for modeskI+G11,kI−G11,kI+G1(−1)andkI−G1(−1), respectively. Colours are defined inb, highlighting different wave vector directions. (b) Multidirectional grating-coupler vectorskin reciprocal space, which have been observed for in-planeHbased onkI. We note that similar combinations with −kIwould be possible. (c) Transmission signal in the BGC with an applied field of 40 mT. Purple and pink dotted lines are calculated for modeskI+G10andkI−G10. The calculated functions are highlighted by the arrows at the graph’s edge. Arrows within the graph highlight related wiggles and fine structures due to avoided crossings, attributed to such BGC modes. (d) Spin-wave resonance frequencies and (e) signal strengths of modes withkI−G01(squares),kI+G01(circles) andkI+G11(triangles) measured on the CoFeB/Py BGCs with different lattice constantsa(θ=90°). All samples are prepared on the same substrate with the same CoFeB thin film. Signal strengths are normalized to thekIsignal. Figure 4: Multidirectional spin-wave detection for different BGCs. ( a ) Data extracted from Fig. 2d for branches highlighted by arrows. Error bars stand for the line width of the resonance. Blue, orange, green and yellow lines are the fittings for modes k I + G 11 , k I − G 11 , k I + G 1(−1) and k I − G 1(−1) , respectively. Colours are defined in b , highlighting different wave vector directions. ( b ) Multidirectional grating-coupler vectors k in reciprocal space, which have been observed for in-plane H based on k I . We note that similar combinations with − k I would be possible. ( c ) Transmission signal in the BGC with an applied field of 40 mT. Purple and pink dotted lines are calculated for modes k I + G 10 and k I − G 10 . The calculated functions are highlighted by the arrows at the graph’s edge. Arrows within the graph highlight related wiggles and fine structures due to avoided crossings, attributed to such BGC modes. ( d ) Spin-wave resonance frequencies and ( e ) signal strengths of modes with k I − G 01 (squares), k I + G 01 (circles) and k I + G 11 (triangles) measured on the CoFeB/Py BGCs with different lattice constants a ( θ =90°). All samples are prepared on the same substrate with the same CoFeB thin film. Signal strengths are normalized to the k I signal. Full size image Considering possible combinations of k I and reciprocal-lattice vectors in Fig. 4b , we realize that modes of k I + G 10 and k I − G 10 have not yet been addressed in the experimental data. SWs with such wave vectors propagate almost in parallel with the CPW. In the reflection configuration used so far, one-and-the-same CPW acts simultaneously as an emitter and detector. As an emitter, the preferential wave-vector direction is transverse to the CPW lines. Similarly, as a detector, a bare CPW reads out transverse wave-vector components preferentially, as the voltage signals induced by a SW plane wave are in phase and add up to a large voltage amplitude. The CPW is not sensitive to ‘longitudinal’ k being parallel to the CPW. This is because in longitudinal direction, all the voltage signals induced by the spin-precessional motion cancel out in the metallic conductor. However, operating two collinear CPWs on the BGC and measuring SW propagation between them in the transmission configuration ( Fig. 1e ), we perceive even such ‘longitudinal’ modes in the propagating SW signals. These modes appear as ‘wiggles’ and signal variations of the ‘transversely’ propagating modes. This is highlighted in Fig. 4c , where we follow the angular dependencies of SW transmission signals through the BGC at 40 mT. The oscillating white–black–white contrast, indicating SW propagation [22] , exhibits regular wiggles and a fine structure indicated by arrows. These features are not observed in propagation measurements on a plane film sample. We attribute such variations of transmitted SW signals to avoided crossings (anticrossings) with coexisting ‘longitudinal’ modes. Avoided crossings are known from plane film studies due to magnon–magnon interaction via dipolar interaction [34] . In Fig. 4c , we show angular dependencies calculated for ‘longitudinal’ modes with k I + G 10 and k I − G 10 (dotted lines highlighted by arrows from outside the graph). Strikingly, the curves go across several of the features indicated by small arrows inside the graph. In Fig. 4b , we summarize the wave vectors of the grating-coupler-induced SWs discussed so far. Importantly, several of the SWs do not propagate in high-symmetry directions of the BGC (for instance, k I + G 11 does not point towards of a 2D square lattice). The magnonic grating coupler thus allows one to send a plane-wave SW in an arbitrary direction simply by adding a tailored CPW-induced k I to the relevant reciprocal-lattice vector, for example, G 11 . Lattice constant and material dependence We provide a quantitative analysis of grating-coupler modes and signal strengths in Fig. 4d,e measured at θ =90°. With increasing lattice constant a , the resonance frequencies measured at k I − G 01 (squares), k I + G 01 (circles) and k I + G 11 (triangles) decrease. As the CPWs exhibited identical geometrical parameters, this is an independent evidence of the grating-coupler effect due to periodic nano-patterning. When we have a larger lattice constant, we create smaller wave vectors |G| . Accordingly, the frequency of the DE mode decreases. The corresponding signal strengths normalized to the k I signal are found to be largest at a =800 nm, that is, at the smallest lattice constant. The grating-coupler-induced SWs with k I − G 01 and k I + G 01 provide spin-precession-induced voltage signals A norm (see Methods section) of almost 20% of the directly excited most prominent mode with k I (fundamental mode). Divided by the intrinsic excitation strength I(k) of the CPW at the relevant wave vector, the relative signal for k I − G 01 is significantly enhanced and amounts to more than η =20,000% ( Fig. 1g and Table 1 ). This value needs to be compared with the intensity of modes at k II and k III , which are at 70 and 90% of the expected relative excitation strength in Fig. 1g . At k I + G 01 , the enhancement η is still about 1,400%. In Fig. 4e , the signal strength for the grating-coupler-induced modes is found to increase with decreasing lattice constant. Magnonic grating couplers with small a are thus most promising. We studied the material dependence of grating-coupler-mode signals in that we fabricated two BGCs with the same geometrical parameters ( a =600 nm) but varied the material composition. We compared CoFeB and Py films with embedded Py and Co nanodisks ( d =305 nm), respectively. Using nominally identical CPWs, we compare the signal amplitudes measured in Im at k I − G 01 normalized to the value Im of mode k I of the same spectrum (red columns in Fig. 5a ). The CoFeB-based BGC provides a considerably larger relative voltage signal. At this point, it is important to realize that for large | k |>| k I |, the measured signal strength underestimates the precessional amplitude of the excited SW. For short-wavelength SWs, voltages cancel, which are induced by out-of-phase antinodes under the central conductor of the CPW (see Fig. 8 in Methods section). As a consequence, only the uncompensated fraction contributes to the measured signal. The blue columns in Fig. 5a provide values that consider the possible compensation due to this purely geometrical effect. For the Py-based BGC, the short-wavelength SW at k I − G 01 reaches ~30% of the amplitude of the fundamental mode with k I . For CoFeB, the mode at k I − G 01 is stronger and reaches ~90%. Its spin-precessional amplitude is thus nearly as large as the fundamental mode at k I . We find of almost 100% for a grating-coupler mode in the CoFeB/Py BGC with a =800 nm (see Table 1 ). Such a large value is similar to conventional optical gratings where higher-order diffraction spots can have the same intensity as the non-diffracted light beam when the openings are small compared with the wavelength. 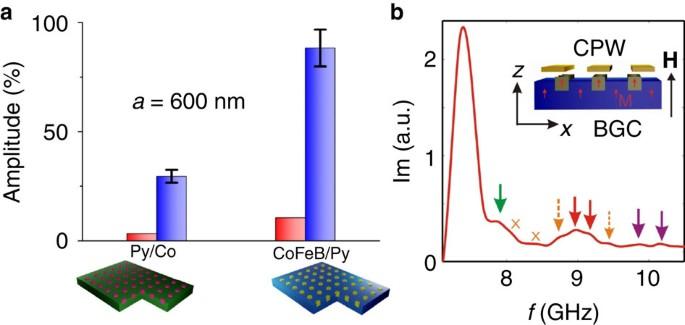Figure 5: Material-dependent coupling and out-of-plane magnetization spin-wave spectra. (a) Material dependence of grating-coupler mode intensities ata=600 nm. Red pillars represent measured voltage signals measured atkI−G01divided by the signal strength observed atkI. Blue pillars stand for the relative precessional amplitude compared with the fundamental mode atkIwhen considering the small wavelength of the spin waves that induces partial cancelation at the CPW (seeFig. 8and Methods section). Error bars are extracted from the unintentional edge roughness of the CPW inner conductor line measured by an scanning electron microscope. (b) Spin-wave reflection spectrum measured on the BGC (a=800 nm) for 1.8 T applied perpendicular to the plane. The orientation ofMis sketched in the inset. The most prominent peak is excited bykI.kIIis contained in thekIpeak. The green arrow indicates thekIIIexcitation. Red arrows indicate the grating-coupler modes ofkI±G01, the orange arrows arekIII±G01modes. Purple arrows showkI±G11modes. Solid (dashed) arrows indicate resonances also seen in in-plane (only in out-of-plane) fields. Crosses mark resonances, which do not shift withH. These originate from the CPW. Figure 5: Material-dependent coupling and out-of-plane magnetization spin-wave spectra. ( a ) Material dependence of grating-coupler mode intensities at a =600 nm. Red pillars represent measured voltage signals measured at k I − G 01 divided by the signal strength observed at k I . Blue pillars stand for the relative precessional amplitude compared with the fundamental mode at k I when considering the small wavelength of the spin waves that induces partial cancelation at the CPW (see Fig. 8 and Methods section). Error bars are extracted from the unintentional edge roughness of the CPW inner conductor line measured by an scanning electron microscope. ( b ) Spin-wave reflection spectrum measured on the BGC ( a =800 nm) for 1.8 T applied perpendicular to the plane. The orientation of M is sketched in the inset. The most prominent peak is excited by k I . k II is contained in the k I peak. The green arrow indicates the k III excitation. Red arrows indicate the grating-coupler modes of k I ± G 01 , the orange arrows are k III ± G 01 modes. Purple arrows show k I ± G 11 modes. Solid (dashed) arrows indicate resonances also seen in in-plane (only in out-of-plane) fields. Crosses mark resonances, which do not shift with H . These originate from the CPW. Full size image SWs for perpendicular magnetization It is now important to investigate the magnonic grating-coupler effect in a perpendicular magnetic field. Perpendicularly magnetized ferromagnetic layers are argued to be advantageous for spintronic nanodevices [35] , [36] , [37] . The same holds true for magnonics where magnetostatic forward volume modes (MSFVMs) follow from a perpendicular-to-plane M . Such MSFVMs can have isotropic in-plane dispersion relations in CoFeB and exhibit, in particular, smaller damping compared with SWs with in-plane M [33] . The in-plane isofrequency contour is a circle similar to the photonic case (black circle in Fig. 1h ). A spectrum taken at a perpendicular field of 1.8 T, being larger than the saturation field of CoFeB, is shown in Fig. 5b . We detect a series of resonances, which we attribute to directly excited and grating-coupler-induced modes (indicated by arrows). The different grating-coupler modes are assigned by calculated MSFVM dispersion relations f ( k ) following ref. 33 . All the arrow-indicated peaks shift to larger frequencies with increasing magnetic field. This behaviour demonstrates that these resonances are due to SWs. Compared with the in-plane field configuration, further higher-order reciprocal-lattice vectors are identified (dashed arrows). From the two last columns of Table 1 , we extract information on how to optimize the magnonic grating coupler for future omnidirectional SW emitters. The filling fraction f ′ matters. The 2D Py/Co BGC has the smallest value f ′ and shows the smallest enhancement η . The 2D ADL and 2D CoFeB/Py BGC have almost the same filling fraction but exhibit very different enhancement η . Introducing ferromagnetic nanodisks leads to a larger signal strength of back-folded modes compared with air holes. In plasmonics, the near field of a metallic grating is used to spatially modulate the far-field electrical field in a coherent manner and couple the radiation to the plasmon [38] , [39] . For magnonics, it is reasonable to assume that the grating-coupler effect originates from a periodic modulation of both the magnetic susceptibility and field, providing the relevant Fourier components at reciprocal-lattice vectors G . Here, the frequency-dependent absolute magnetic susceptibilities of the BGC components enter. We attribute the different signal strengths of Fig. 5a to the different susceptibilities of the periodic scattering centres, that is, the nanodisks made either from Co or Py. At the same time, we expect the dynamic stray fields from the periodically patterned film to be relevant [40] , making the observed enhancement effect particularly material dependent. Following this, the precessional amplitudes of back-folded modes depend on both the individual magnetic susceptibilities and magnetic contrast between the materials forming the BGC. For optical transmission gratings, if one wants to detect higher orders in the diffraction pattern, one should make the openings as small as possible, approaching a δ -function. Therefore, if one decreases the nanodisk diameter, higher-order modes such as k I ±2 × G 01 and k I ±3 × G 01 might become visible. We indeed observe such modes in the 2D Py/Co BGC with the smallest nanodisk filling f ′=0.15 in in-plane fields. We extract modes with large reciprocal-lattice vectors for a 2D BGC with a slightly larger f ′=0.22 also in out-of-plane fields ( Fig. 5b ). We attribute this latter observation to the more homogeneous internal field [41] and the superior damping in CoFeB for perpendicular M (ref. 42 ). Besides the periodic square lattice investigated here, there exist four more Bravais lattices of different symmetry in 2D, which allow for more magnonic grating couplers with SW emission in further spatial directions. The formalism of ref. 40 suggests a 1/(1+2 r / d ) 2 dependence for the rf field enhancement near a columnar magnetic scatterer ( r is the distance from the edge of the magnetic scatterer). This dependence explains qualitatively the observed signal increase with decreasing a at fixed diameter d of nanodisks in Fig. 4e . A smaller lattice constant a means that the intermediate CoFeB resides at smaller r in average. The reduced a thereby enlarges the rf magnetic field components originating from neighbouring nanodisks and acting on the CoFeB in between. Making use of resonant magnetic scattering [40] , we expect even larger enhancements η than reported here. For an individual BGC, an emitted wave is, in particular, a plane wave being important for parallel processing in CNNs. A hexagonal lattice of nanodisks might provide both the largest spin-precessional amplitudes and, for out-of-plane fields, SW emission into the largest number of equivalent in-plane directions. Combinations of different BGC lattices underneath a single CPW now allow one to provoke omnidirectional SW emission from straight antennas. In contrast to the ideal ‘omnidirectional antenna’ discussed for electromagnetic waves in free space, the SW amplitude is expected to vary in different directions. In plasmonics, grating couplers with complex designs have opened the field of wave-front engineering for, for example, focussing devices [23] . Similar developments are expected for magnonics [28] . Here, the reprogramming of periodic magnetic states [43] , [44] , [45] , [46] is particularly intriguing and opens novel perspectives such as reprogrammable grating couplers and focusing. The maximum wave vector k (minimum wavelength) obtained with magnonic grating couplers in Table 1 amounts to about 18 rad μm −1 (350 nm), being a factor of 5 and 720 larger (smaller) compared with the wave vectors (wavelengths) excited very recently by all-optical methods in refs 18 , 19 . Compared with the free-space electromagnetic wave at the same f , we reduced the SW wavelength by more than four orders of magnitude. Smaller lattice constants a <600 nm prepared by state-of-the-art nanolithography will allow one to achieve even larger | k |, that is, SW wavelengths λ <350 nm by means of magnonic grating couplers. Such small λ might not be achieved by light due to the diffraction limit. The couplers are thus powerful for different nanotechnologies such as CNNs and phase control of STT–NOs. Thinking of networks of STT–NOs [35] , [47] , [48] , the straight phase fronts of grating-coupler-induced SWs are expected to coherently control the phase in specific rows of one-and-the-same array of STT–NOs as sketched in Fig. 6 . Pufall et al . [15] demonstrated that SWs rather than magnetic fields are the primary interaction mechanism for phase locking between two neighbouring NOs in their experiments. Phase locking of NOs is the key, for example, for large microwave power levels extracted from NO arrays and information processing with SWs [14] . In Fig. 6 , we propose a spintronic device that uses grating-coupler-induced SWs to phase-lock NOs. This approach may answer to the remaining challenge of reconfigurable phase control in a large NO array for information processing. The spatial orientation of a front of constant SW phase can be selected specifically by an appropriate G via the frequency at the clock CPW. Making use of a different G modifies the rows of NOs experiencing the same SW phase. This feature goes beyond an individual NO used for phase control of neighbouring NOs. Magnonics has been shown to support data processing in a non-reciprocal way [49] . The non-reciprocity is already seen in transmission spectra (see Fig. 7c in Methods section) where branches exhibit different signal strengths for H <0 and H >0. The magnonic grating-coupler effect presented here thus allows for non-reciprocal phase control of arrays of STT–NOs. 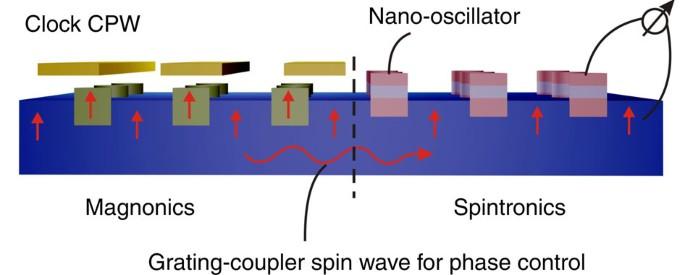Figure 6: Proposed device in magnon spintronics. Sketch of the proposed device interconnecting magnonics and spintronics. It is based on grating-coupler-induced spin waves (horizontal curved arrow) excited by a clock CPW (left) for the phase control of an STT-NO array (right). Straight arrows indicate the magnetization orientation. Figure 6: Proposed device in magnon spintronics. Sketch of the proposed device interconnecting magnonics and spintronics. It is based on grating-coupler-induced spin waves (horizontal curved arrow) excited by a clock CPW (left) for the phase control of an STT-NO array (right). Straight arrows indicate the magnetization orientation. 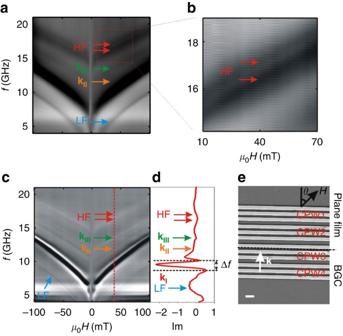Figure 7: Field-dependent spin-wave spectroscopy and scanning electron microscope (SEM) image of a BGC. (a) Grey-scale plot of spectra taken in reflection configuration on CPW4. The fieldHis collinear with the CPW (θ=90°). Arrows indicate modeskI,kIIandkIII, as well as LF and HF modes. A zoom-in image is shown inb, where we adjust the figure contrast to highlight the two HF modes. (c) Imaginary part (Im) of spectra taken in transmission configuration, where spin waves are excited at CPW4 and then detected at CPW3, both residing on the BGC. The dashed line is at 40 mT where we extract the individual spectrum shown ind. The frequency separation denoted by Δfis used to calculate the group velocity. (e) SEM image of the CoFeB/Py sample adjacent to a plane-film part where we label the CPWs and defineθ. Scale bar, 5 μm. Full size image Figure 7: Field-dependent spin-wave spectroscopy and scanning electron microscope (SEM) image of a BGC. ( a ) Grey-scale plot of spectra taken in reflection configuration on CPW4. The field H is collinear with the CPW ( θ= 90°). Arrows indicate modes k I , k II and k III , as well as LF and HF modes. A zoom-in image is shown in b , where we adjust the figure contrast to highlight the two HF modes. ( c ) Imaginary part (Im) of spectra taken in transmission configuration, where spin waves are excited at CPW4 and then detected at CPW3, both residing on the BGC. The dashed line is at 40 mT where we extract the individual spectrum shown in d . The frequency separation denoted by Δ f is used to calculate the group velocity. ( e ) SEM image of the CoFeB/Py sample adjacent to a plane-film part where we label the CPWs and define θ . Scale bar, 5 μm. Full size image We note that the BGC might enable one to directly detect ‘longitudinal’ modes, not possible with a bare CPW. From plasmonics, it is known that bi-gratings provide efficient coupling of short-wavelength surface plasmons from all in-plane directions to the long-wavelength light radiation [32] , [50] . In an analogous way, a CPW prepared on top of a BGC forms a magnon-to-microwave transducer for SWs from different in-plane directions. Its efficiency is yet to be explored. In our device, the detected microwave signal is expected to be vanishingly small as the effective propagation length for the excited ‘longitudinal’ modes amounts to ~100 μm from the emitter to detector signal line. A mode k I + G 10 leaves the emitter under a shallow angle of φ =6.7° giving rise to a propagation length of s /sin φ =103 μm with s =12 μm. This value is larger than the decay length in CoFeB [42] . 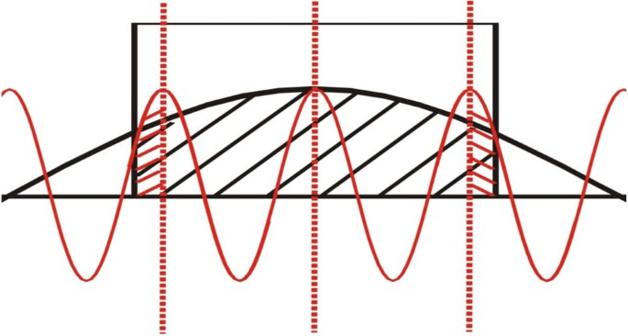Figure 8: Calculation of effective spin-precessional amplitudes. The black curve is the wave form of modekIwith a wavelength of 6,830 nm. The red curve is an example for a grating-coupler mode with a much shorter wavelength. The vertical black lines indicate the outer boundary of the inner conductor of the CPW that picks up the spin-precession-induced voltage. The hatched areas are assumed to be effective for voltage induction. Figure 8: Calculation of effective spin-precessional amplitudes. The black curve is the wave form of mode k I with a wavelength of 6,830 nm. The red curve is an example for a grating-coupler mode with a much shorter wavelength. The vertical black lines indicate the outer boundary of the inner conductor of the CPW that picks up the spin-precession-induced voltage. The hatched areas are assumed to be effective for voltage induction. Full size image Compared with STT–NOs as SW emitters, the investigated nanograting method does not require electrical contacts to nanopillars, and can generate plane waves with straight phase fronts in both in-plane and out-of-plane fields, which is essential for multibranch SW logic devices. The nanograting method can be directly integrated on a chip via lithography [51] and is thus more compact compared with light-generated SWs where optical micro lenses are required and adjusted to exact positions. Extra damping by magnon scattering is expected in in-plane fields only for selected frequencies when G vectors connect dispersion relations in different spatial directions at the same frequency [52] . For the out-of-plane field configuration, this issue is not relevant, thanks to the modified dispersion relations [53] . In conclusion, changing the magnetic contrast between two materials and the geometrical parameters of BGCs, the grating effect supports omnidirectional emission of SWs using straight and compact microwave antennas. We observe short-wavelength DE modes in many spatial directions, decided by the field orientation θ and the microwave frequency. Plane waves from magnonic grating couplers exhibit a stable phase excited by the microwave generator. The stable phase is relevant for operating CNNs. Notably, the magnonic grating coupler works without restrictions in both in-plane and out-of-plane fields. This goes beyond NOs where the field orientation needs to be specifically optimized. Our findings on microwave-to-magnon transducers pave the way for the development and advancement of SW-based electronics and magnon spintronics. Sample fabrication The CoFeB/Py BGC is fabricated as follows. First, a CoFeB thin film is prepared on a semi-insulating gallium arsenide substrate by magnetron sputtering in a Xenon atmosphere using a Co 20 Fe 60 B 20 target. The thin film forms a mesa with an area of 150 μm × 100 μm, defined by the optical lithography mask. The thickness of the film is measured with an atomic force microscope. Second, using electron-beam lithography (EBL), we prepare a resist mask with a periodic square lattice of holes and then use Ar ion milling to etch nanotroughs into the CoFeB thin film. Without taking the sample out of the vacuum chamber, we refill the nanotroughs with Py using electron-beam evaporation. Third, a 10-nm thick layer of Al 2 O 3 is grown by atomic layer deposition onto the mesa to ensure an electrical isolation for the metallic CPWs. Finally, CPWs are integrated by EBL, and electron-beam evaporation of gold for both signal and ground lines. Each line is 2.1 μm wide. The edge-to-edge separation between signal and ground lines is 1.5 μm. The distance s between the two signal lines of neighbouring CPWs is 12 μm. The Py/Co BGC is fabricated in the same way, except that both Py and Co are deposited by electron-beam evaporation. The one-dimensional BGC is prepared from periodic Py nanowires patterned by EBL and lift-off processing, and then covered with a sputtered CoFeB thin film. The 2D ADL is fabricated by first creating a Py thin film mesa with optical lithography and then etching a 2D periodic nanotrough array into the film using Ar ion milling. All-electrical SW spectroscopy Using micropatterned CPWs and a 4-port VNA, a broadband SW spectrometer has been set up to explore collective spin excitations in an all-electrical approach. It covers the frequency range from 10 MHz up to 26.5 GHz. The power used in the experiments is 0 dBm. The CPW provides both the microwave field excitation and the detection of SWs. The detected voltage is induced by the precessing spins. The CPW is integrated on the top of the devices as the last step of the sample preparation. The samples are located between current-carrying coils, which generate a DC magnetic field H for field-dependent measurements. H is applied in different spatial directions. The SW wave vectors excited directly by the CPW can be calculated by Fourier transformation of the dynamic magnetic-field distribution. Using the lateral dimensions of the CPW, that is, line widths of signal and ground lines, as well as edge-to-edge separations, we calculate the spatial distribution of the dynamic magnetic field. After a Fourier transformation, we derive the excitation intensity for different k , in Fig. 1g , where we have first, second and third excitations at k I , k II and k III , respectively. The values are | k I |=0.92, | k II |=2.75 and | k III |=4.85 rad μm −1 . The effective magnetization of CoFeB is measured to be 1.52 T. When the applied field is rotated from 90° to 0°, for instance, the SW dispersion relation (frequency f versus k ) transforms from a pure DE mode of large frequency with a positive group velocity v g to a BVMSW mode of low frequency (LF) with negative v g , respectively, at small k . This anisotropy is a special feature of magnons in contrast to photons. For angles between 90° to 0°, the dispersion relation is a combination of both mode types. Considering this and following refs 31 , 33 , we modelled the angular-dependent SW excitations. Considering the grating-coupler-induced modes, an additive reciprocal-lattice wave vector G is provoked by the Fourier components provided by the periodic patterning such as G 01 , G 10 and G 11 . For k I ± G 01 , the absolute value of the wave vector is varied but not the orientation; therefore, the SW modes fall on the original dispersion relation being relevant for the k I direction. However, for k = k I ± G 10 (or k = k I ± G 11 ), the wave-vector direction differs from k I , and maximum resonance frequencies attributed to the DE mode configuration of M perpendicular to k occur at different angles θ compared with k I . Field-dependent measurements Figure 7 shows field-dependent spectra taken on the CoFeB/Py BGC in reflection and transmission configurations and a scanning electron microscopy image showing four separate CPWs on one-and-the-same thin-film sample. Two of them reside on the BGC. The further two CPWs are on an adjacent plane-film area (unpatterned). In Fig. 7a , we show spectra in reflection configuration taken on CPW4 with θ =90°, that is, H is parallel to the CPW lines. Thus, k I is perpendicular to M and we study the DE-type SWs [33] . The most pronounced mode is generated by the CPW at k I . The second mode at k II is relatively weak and above the k I mode. We clearly observe the mode with k III between 12 GHz and 16 GHz. These three modes are also observed on CPW1 and CPW2 on the plane-film area (data not shown). Interestingly, there are additional modes detected exclusively on the BGC but not in the plane film. Two are the HF modes that appear between 15 GHz and 20 GHz, and the other one is a LF mode between 4 and 10 GHz. This LF mode is consistent with a mode studied by Duerr et al . [10] in a Py/Co MC and will not be discussed here, as its nature is already known. We focus on the HF modes. In Fig. 7b , we adjust the contrast to have an optimized view on the HF modes, substantiating two separate modes close to each other (arrows). They obey a similar field dependence. The frequency separation amounts to about 1.2 GHz. Figure 7c contains the Im part of the transmission signal taken between CPW3 and CPW4. Considering the pronounced white–black–white oscillating contrast, a clear SW propagation signal is found for the mode at k I . The large oscillation seen in the spectrum ( Fig. 7d ) allows us to extract the SW group velocity [22] , using Δ f and =Δ f·s =18 km s −1 . Here, s =12 μm is the propagation distance between emitter and detector CPWs. The value v g is consistent with SW group velocities found in an unpatterned CoFeB thin film [42] . In Fig. 7c , weak transmission signals are seen for k III and both HF modes as well. Around the mode at k III , we see an interesting asymmetry in the transmission signal for H <0 and H >0. We explain this asymmetry by grating coupler modes, that overlap with each other and exhibit different signal strengths depending on the field orientation due to non-reciprocal excitation [48] . Calculation of spin-precessional amplitudes In Fig. 8 , we introduce the method of calculating the relative spin-precessional amplitude of a short-wavelength SW compared with the spin-precessional amplitude of the fundamental mode at wave vector k I . For this, one needs to consider the finite width of the CPW conductors, the SW wavelengths λ and the different excitations frequencies f . First, we read out the measured signal where we take the height of a BGC SW resonance peak ( S BGC ) in Im ( c.f. , Figs 2a and 5b ) at resonance frequency f ( k ). Second, we normalize this value to the signal strength extracted for the k I mode ( ) of one-and-the-same spectrum (see Fig. 2a ) by . We depict this normalized value A norm as a red pillar in Fig. 5a . Values A norm are also plotted in Figs 1g and 4e . Considering the grating-coupler mode with k I − G 01 at a =800 nm, we calculate the wavelength λ to be 658 nm, which is much shorter than that of the k I mode being about 6,830 nm. We compare the two wavelengths in Fig. 8 with the width of the central conductor of the CPW. Here we assume that the sensing area of the CPW is given by the geometrical width of the metallic conductor (indicated by an area hatched in black colour) that picks up the spin-precession-induced voltage. On the one hand, we see that for the grating-coupler mode with small λ (red full line), several π -phase-shifted antinodes are out of phase and induce counteracting voltage signals in the metallic conductor. As a consequence, most part of the oscillation cancels out. Only the region E eff (hatched in red colour) is effective for the induced voltage signal. On the other hand, for the k I mode the spin-precessional motion is in-phase throughout the metallic conductor and the signal is produced by the region E sens hatched in black colour. E eff / E sens is a factor describing the direct detection efficiency of the CPW for a SW with a given λ , neglecting a transducer effect of the BGC. The cancellation mechanism can also explain that some modes are visible in some sample, but might disappear in some other sample with slightly different CPW widths or lattice constants. At some particular wavelength, the measured signal may be zero if a full SW wavelength fits into the width of the CPW. As the time-derivative d M / dt of the magnetization M enters the voltage induced in the metallic conductor, the relative spin-precession amplitude needs to consider this according to: . This equation provides the relative measure of the spin-precessional amplitude at k I − G 01 compared with the fundamental-mode amplitude at k I . We depict the value as a blue pillar in Fig. 5a . As we can see from the red shaded area in Fig. 8 , the effective excitation of grating-coupler mode is sensitive to the edges of the inner conductor of the CPW. From the scanning electron microscope image, we extract an edge roughness of ±14 nm. This roughness leads to an error bar of the calculated value , plotted in the Fig. 5a . Simulation of SW modes with angular dependence From refs 31 , 33 , we model the angular-dependent SW excitations. The following equations (1) and (2) show the dispersion relations for DE and BVMSW modes, respectively, where ω H = γμ 0 H , ω M = γμ 0 M s ; d stands for the thickness of the film and M s is the saturation magnetization: By combining these two equations, we calculate the dispersion at any angle in between ( Fig. 3 ). At a specific wave vector k , we extract the resonance frequencies as a function of θ by drawing a vertical line at a given k -value and searching for the crossing points with different dispersion relations f ( k , H , θ ) (see Fig. 3 ). Such frequency variation with θ are plotted as lines in Figs 2b,d and 4a,c . How to cite this article: Yu, H. et al . Omnidirectional spin-wave nanograting coupler. Nat. Commun. 4:2702 doi: 10.1038/ncomms3702 (2013).